Simulation of non-Abelian gauge theories with optical lattices Many phenomena occurring in strongly correlated quantum systems still await conclusive explanations. The absence of isolated free quarks in nature is an example. It is attributed to quark confinement, whose origin is not yet understood. The phase diagram for nuclear matter at general temperatures and densities, studied in heavy-ion collisions, is not settled. Finally, we have no definitive theory of high-temperature superconductivity. Though we have theories that could underlie such physics, we lack the tools to determine the experimental consequences of these theories. Quantum simulators may provide such tools. Here we show how to engineer quantum simulators of non-Abelian lattice gauge theories. The systems we consider have several applications: they can be used to mimic quark confinement or to study dimer and valence-bond states (which may be relevant for high-temperature superconductors). Gauge theories (GTs) [1] provide the basis of modern physics. In the standard model of particle physics [2] , GTs describe three of the four fundamental interactions (namely electromagnetic, weak and strong interactions). The last is described by the GT known as quantum chromo-dynamics (QCD) [3] ). Gauge symmetry has also a role in general relativity. At the same time, GT are present in many effective models of condensed matter, for example, antiferromagnets [4] and high-temperature superconductors [5] , [6] . Recently, the study of phase diagrams of various GT has gained new attention, because of the discovery of topological order. Owing to their stability against perturbations, topologically ordered phases may help to design quantum computers [7] , [8] , [9] , [10] , [11] . Despite the enormous importance of GT, they defy solution. Wilson’s formulation [12] of lattice gauge theories (LGTs), where continuous space–time is replaced by a discrete set of points, provided the first numerical tool to study the strong-coupling regime. Monte-Carlo (MC) simulations of LGT is the main tool to compare aspects of QCD at strong coupling with experiments [13] . What is hard or impossible to compute with MC remains out of reach. For example, the mechanism of charge confinement [14] , invented to explain the absence of isolated quarks [15] , is still debated four decades since first proposed. Furthermore, MC simulations cannot yet provide definite predictions for hot and dense nuclear matter [16] , [17] , probed by heavy nuclei collisions at CERN and RHIC [18] , [19] . GT are also invoked in explanations of spin-liquid phases of antiferromagnets [4] and high-temperature superconductivity [20] . Recent progress in the experimental control of quantum systems makes possible to engineer systems that perfectly mimic theoretical models. This is the idea of quantum simulators [21] , [22] , [23] , [24] , [25] , [26] , whose ultimate goal is to simulate GT, for example, QCD,and provide access to their phase diagrams at finite temperature and density. A more modest goal is to emulate QCD, that is, to find a model sharing its interesting properties, whose realization may be simpler than the full theory. The first steps of this emulation programme were to describe quantum simulations of Abelian LGT [27] , [28] , [29] , [30] , [31] , [32] . The presence of many-body interactions, beyond nearest neighbours, has been the main technical obstacle. This obstacle has been addressed in [29] , by using mesoscopic Rydberg gates [33] . Here we show how to simulate non-Abelian gauge magnets (GMs) or link models, introduced in (refs 34 , 35 , 36 ) using Rydberg atoms [37] , [38] . The models have both strong- and weak-coupling regimes. We discuss here the origin of charge confinement in both regimes, stressing the different physical origin in each. We propose how to identify the flux tubes connecting static external charges in each of these regimes, and provide the experimental protocol to observe these flux tubes. We conclude by discussing a qualitative technique, based on energy landscapes around static charges, to identify in a generic LGT whether chromo-electric strings, that is, charge confinement, is present. The model Here we want to analyse a specific non-Abelian GT that can be simulated with ultra-cold atoms. GTs were originally introduced in the context of relativistic field theories as generalization of quantum electrodynamics (QED), the theory of photons and electrons, and hence formulated through a Lagrangian density that does not distinguish between space and time. In order study them with quantum simulators, we need their Hamiltonian formulation [39] , [40] on the lattice. There, the constituents representing the gauge bosons (generalization of photons) live on the links of the lattice and those representing the charged matter (generalization of electrons) live on the sites. The Hamiltonian of a LGT is manifestly invariant under a group of local transformations. These transformations encode the generalization of the Gauss law, that physically enforces the charge conservation. The choice of the symmetry group determines if we are dealing with an Abelian (for example, QED) or non-Abelian LGT. One of the simplest non-Abelian LGT is the SU(2) LGT. The specific form of the Hamiltonian and the Hilbert space of the constituents determines which SU(2) LGT one considers. The standard SU(2) LGT, called Yang–Mills (YM) theory, involves an infinite dimensional Hilbert space for the gauge bosons and an Hamiltonian obtained directly from the original Wilson action [12] . In a quantum simulation, we encode the states of the constituents in hyperfine levels of the atoms. For this reason, we want to study first the simplest SU(2) LGT having as small as possible local Hilbert space. This leads to the family of the SU(2) GM. Although their physical properties are quite different from the one of the YM theory, the SU(2) GM we analyse here shares with YM theory the phenomenon of confinement of charges. In the following, we briefly motivate the construction of these models but we invite the reader interested in obtaining a deeper understanding to directly refer to either the original papers [34] , [35] , [36] or to the existing reviews on the subject [29] , [41] . In the SU(2) GM, gauge bosons have four states, so that their Hilbert space is isomorphic C 2 ⊗ C 2 . In order to impose the Gauss law, we first need to define the operators that implement the rotation of an arbitrary group element. An element of SU(2) can be written as exp[ i α · σ ] where α =( α 1 , α 2 , α 3 ) is the real three-component vector and σ =( σ 1 , σ 2 , σ 3 ) are the Pauli matrices. The rotation of a link state through a group element is obtained with the two operators In this way, we can define a local transformation in the absence of external charges as on the crosses, which consist of the four spin states adjacent to given site s (labelled s 1 ,…, s 4 ; see Fig. 1b ). The operators are unitary, fulfil Ξ( α 1 )Ξ( α 2 )=Ξ( α 1 α 2 ), so to provide a representation of SU(2), and only act locally. We thus identify them as a set of local symmetry transformations. 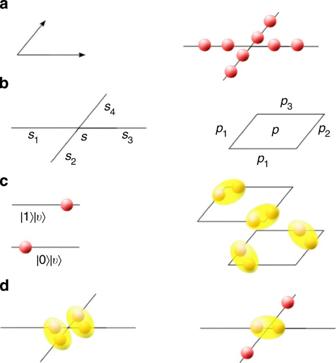Figure 1: The basics of non-Abelian GM. (a)Hilbert space, we assign to each link of an oriented lattice (left), the Hilbert space of two qubits, each of them represented by a sphere (right). (b) Notation, a link may be labelled in either of two equivalent ways: by adding a subscript referring to the adjacent site (left panel), or to the adjacent plaquette (right panel). We number these labels anticlockwise. (c) Physical interpretation, representation of position and spin degrees of freedom, a red sphere on the left of a link represents the state, whereas a red sphere on the right of a link represents the state(left panel). Gauge-invariant space for a plaquette, gauge-invariance forces qubits adjacent to a site to form singlets (yellow ovals around them) (right panel). (d) Gauge-invariant states, example of gauge-invariant state for a generic lattice. The gauge-invariance constraint, having the role of the QED Gauss law, selects those states invariant under the above local symmetry transformations, Figure 1: The basics of non-Abelian GM. ( a )Hilbert space, we assign to each link of an oriented lattice (left), the Hilbert space of two qubits, each of them represented by a sphere (right). ( b ) Notation, a link may be labelled in either of two equivalent ways: by adding a subscript referring to the adjacent site (left panel), or to the adjacent plaquette (right panel). We number these labels anticlockwise. ( c ) Physical interpretation, representation of position and spin degrees of freedom, a red sphere on the left of a link represents the state , whereas a red sphere on the right of a link represents the state (left panel). Gauge-invariant space for a plaquette, gauge-invariance forces qubits adjacent to a site to form singlets (yellow ovals around them) (right panel). ( d ) Gauge-invariant states, example of gauge-invariant state for a generic lattice. Full size image which are the only physical states of the LGT. It is sufficient to impose this condition for α equal to =(1, 0, 0), =(0, 1, 0) and =(0, 0, 1). We can derive the physical consequences of equation (4). We interpret the local Hilbert space as , describing one qubit (the right factor, ) moving between the two ends of the link (the left factor, ). We identify the basis of , and , with the left-end (lower end) or the right end (upper end) of a link in the x ( y ) direction. In this way, given a generic state in , we represent as a solid dot on the left (right) part of the link, cf . Fig. 1c ). The operator Ξ( α ) acts on those vectors in the left (down) two-dimensional subspace of the x ( y )-oriented link (rotating them by exp( i α · σ )). The operator ( α ) acts similarly on the other subspace of that link. Hence, the physical-state condition (4) forces the total spin of the qubits adjacent to the site s to be zero, that is, to consists of singlet among pairs of those, , cf . Fig. 1d ). Charges are encoded by additional qubits on the sites of the lattice. Different spin representations S =1/2, 1, 3/2, 2 require the addition of a different amount of qubits. The presence of charge at the site implies that the gauge transformations at induce a rotation of the state Here we focus on the case of spin-1/2 charges, that is, S ≡ σ . In this case, the charge is encoded by a qubit located at and equation (5) can be expressed as follows: with . We now turn to the form of the Hamiltonian H . We built H as a sum of plaquette, H p , and link, H l , operators as for ordinary LGT ( p and l label the plaquettes and the links of the lattice). The former corresponds to the magnetic term ( B 2 in electrodynamics), whereas the latter is the analogue of the electric term ( E 2 ). A convenient set of operators to write H p and H l is (see ref. 35 ) Gauge invariance, that is, [ G s , H ]=0, ∀ s , fixes H l and H p . It immediately implies [Ξ( α ), H l ]=0, thus, H l Γ 5 (plus trivial identity term). H p can be written as tr V ( U p 1 ⊗ U p 2 ⊗ U p 3 † ⊗ U p 4 † ), p 1 ,… , p 4 being the links around the plaquette p , ordered as in Fig. 1b ). At each link, the U acts on ( ), where V is an auxiliary bookkeeping spin-1/2 space on which the trace is performed. V is not physically implemented in the simulator and is introduced only to write covariant expression easily. The gauge-invariance requirement for U reads where τ j , j =1, 2, 3 is a Pauli matrix on V . Again, equation (8) has the same form as in standard LGT. A solution of equation (8) is , that is, the one we consider here. Thus, where Δ is an energy scale. The coupling constant g determines if the system is in the weak- or in the strong-coupling regime ( g →0 and g →∞, respectively). The confinement phase The phases of LGT are commonly characterized through the force induced by gauge bosons on the charges. Here we are interested in studying the confinement phase, that is, the phase where the attractive force between two charges, does not depend on their distance. In this case, the ground state energy of the system in the presence of two charges, increases linearly with their separation. At weak coupling, H in equation (9) reduces to its plaquette terms. In analogy with the Abelian case [29] , we exploit the bi-partite nature of the lattice. We imagine colouring the plaquettes red and black in a checker-board pattern. Next we consider the Hamiltonian equation (9), but including only half the terms, for example, those on the black plaquettes. With this choice, the model becomes exactly solvable. As illustrated in Fig. 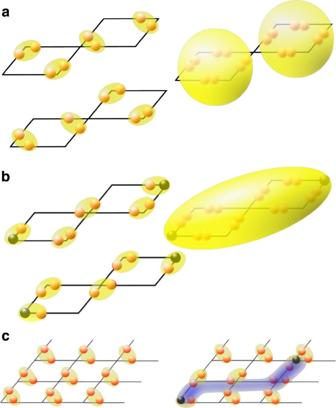Figure 2: Confinement of charges. (a,b) Weak coupling. (a) In the absence of external charges, dimers resonate on configurations allowed by gauge invariance. (b) When two static charges (black spheres) are inserted, plaquettes are entangled by strings of singlets. In this way, a macromolecule or polymer, as large as the separation of the charges, is formed (yellow oval). The energy of such a state rises linearly with the inter-charge separation, thereby confining charges. (c) Strong coupling. The ground state of equation (9) is the ordered configuration where all position qubits are in the stateand spin qubits are forced by equation (4) to form singlets (left panel). When two external charges are inserted (black spheres), the singlets have to rearrange (right panel). Some of the position qubits are flipped towith an associated energy cost. Pictorially the corresponding spin qubits shift right-up on thex–ylinks. A string can be identified by position qubits in state. The energy cost of a string is proportional to its length, hence, the charges are confined. 2a ), the ground state is a product state of single plaquette configurations, Figure 2: Confinement of charges. ( a , b ) Weak coupling. ( a ) In the absence of external charges, dimers resonate on configurations allowed by gauge invariance. ( b ) When two static charges (black spheres) are inserted, plaquettes are entangled by strings of singlets. In this way, a macromolecule or polymer, as large as the separation of the charges, is formed (yellow oval). The energy of such a state rises linearly with the inter-charge separation, thereby confining charges. ( c ) Strong coupling. The ground state of equation (9) is the ordered configuration where all position qubits are in the state and spin qubits are forced by equation (4) to form singlets (left panel). When two external charges are inserted (black spheres), the singlets have to rearrange (right panel). Some of the position qubits are flipped to with an associated energy cost. Pictorially the corresponding spin qubits shift right-up on the x – y links. A string can be identified by position qubits in state . The energy cost of a string is proportional to its length, hence, the charges are confined. Full size image where S p 1, p 2 S p 3, p 4 and . We separate the position part of the Hilbert space from its spin part by writing the states as elements of ⊗ 4 ⊗ ⊗ 4 . Both and are represented in Fig. 1c ). The state factorizes into resonating-dimer states. Furthermore, each link, as a consequence of gauge invariance, is entangled with the rest of the system. We now turn to confinement. Adding a pair of spatially separated external charges rearranges the singlets into strings connecting the charges. Each string causes long-range entanglement (LRE) between the charges, a distinctive feature of non-Abelian LGT. In an Abelian LGT, indeed, a single string does not induce entanglement, as typically it involves flipping a line of spins [42] . There, the unique source of LRE between charges is caused by the linear superposition of several orthogonal string states, present also here. The ground state is indeed a superposition of string states along paths determined by both gauge invariance and energy minimization. A string passing through a plaquette increases its energy by δE Δ/ g . Hence, strings touch as few plaquettes as possible. The number of excited plaquettes is proportional to the inter-charge distance, that is, the charges are confined with a string tension proportional to Δ/ g . This phenomenon is equivalent to the chromo-electric flux tube expected in QCD between two coloured charges. The simplest system exhibiting such behaviour consists of only two plaquettes ( Fig. 2b ). At strong coupling, the plaquette term in equation (9) may be neglected. The ground state is the configuration with all the position qubits in the state . Hence at any site s , the spin qubits on s 3 , s 4 form a singlet, see Fig. 2c left. This is a product state of entangled half-plaquettes, of the form . If we now insert two static charges, a line of singlets must readjust. As consequence of equation (6), the two spin qubits , , originally forming the singlet at , rearrange. One qubit, say forms a singlet with the external charge, whereas the position state associated to the other qubit changes from to , that is, the qubit moves to the opposite end of the link. There, by equation (4), it is forced to form a singlet with one of the two qubits of the same cross. The process repeats until one of the displaced qubits reaches the second external charge. The result is a gauge-invariant string, stretching between the charges. The string is a line of qubits in state . The energy of each of them increases by 2Δ; therefore, the static charges are confined. Note that the the actual ground state is a superposition of orthogonal strings states inducing LRE between the external charges. However, each single string already entangles the two charges, footprint of a non-Abelian LGT. Realization through Rydberg atoms We implement the SU(2) GM using cold atoms loaded in an optical lattice. We start by describing a generic scheme that works for arbitrary values of g , and then consider a simplified scheme suited to study the g →∞ limit. Generic scheme . We distinguish two cases. (i) The pure GT where atoms only encode the gauge boson degrees of freedom on the links and (ii) gauge fields interacting with matter, where we need extra atoms to encode the charges at the sites. We generically refer to all these atoms as ensemble atoms. As all local Hilbert spaces are tensor product of qubits, each of them is represented by two (long-lived) hyperfine states of one atom. The Hamiltonian (equation (9)) and symmetry projections operators (equation (4)) act on at least eight neighbouring atoms. We engineer both sets of operators using the mesoscopic Rydberg gates [33] , [37] . The idea is to add an auxiliary two-level system as a control atom. The control acts as a switch that turns on and off the interaction between the ensemble atoms, that is, simultaneous Rabi transfer (SRT) between two hyperfine levels of each of the atoms. Such operations are induced by laser pulses. In practice, when the control is initialized in the logical state nothing happens, while, once initialized in , the control is excited to a specific Rydberg state, and causes SRT on the ensemble atoms within its blockade radius. The operators in both equations (9) and (4) can be decomposed in linear combination of these SRT (see below and Methods). As we only use internal degrees of freedom, the atoms are assumed to be frozen in a Mott state. Note that the (Zeeman) energy splitting between the logical states (which can be controlled with a magnetic field) and the lattice depth (controlled by laser intensity) can be taken sufficiently large to minimize imperfections due to the temperature of atomic sample (see Methods). In fact, for ideal gates the simulated temperature of the GM would be zero. Thus, the requirements for the implementation of eqautions 4 and 9 through Rydberg gates are: (a) deep optical lattice loaded with (b) two ensemble atoms per link, that is, the four states of the gauge boson, and with the appropriate number of matter atoms at each site; (c) one control atom for each cross (at each site) and plaquette (inside it); (d) both ensemble and control atoms have two logic (sufficiently split hyperfine) states that can be excited to (different) Rydberg states by laser pulses; (e) the lattice spacing should be tuned such that the ensemble atoms of crosses and plaquettes are physically located inside the blockade radius of their respective control. One way to obtain the desired optical lattice for both (i) and (ii) is sketched in Fig. 3a,b , respectively, is to use holographic techniques [43] . In Fig. 3a , atoms are represented as spheres, ensemble atoms are red and control atoms are blue. The required blockade radii are indicated by shaded regions in cyan and orange. In presence of matter, a possible lattice configuration is shown in Fig. 3b . Effective sites (shaded in green) now involve four atoms. Three of them encode the charges (black), whereas the fourth is a control atom (blue). Links (shaded in green) connect these effective sites. Again the desired blockade radii are represented by shaded regions, cyan for crosses and yellow for plaquettes. 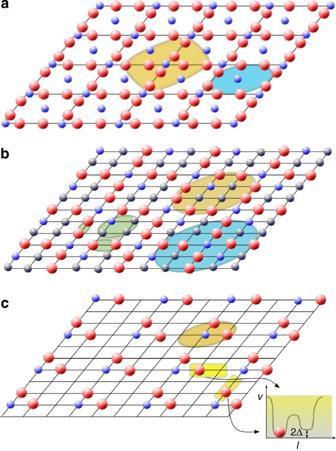Figure 3: Lattices of Rydberg atoms needed for simulating SU(2) GM. (a) Holographic lattice scheme for the simulation of the pure LGT at weak coupling. Blue spheres represent the control two-level atoms, whereas red spheres are the ensemble two-level atoms. The blockade radii for a plaquette-control atom and the cross-control atom are shaded in cyan and orange, respectively. (b) A different lattice scheme has to be used to introduce static charges. It is made from super-sites including four two-level atoms (shaded green circle). One of these is a cross-control atom (blue), whereas the other three are used to encode static charges (black). The links of the gauge magnets, which connect these effective sites, have two atoms each (red spheres on shaded green oval). Atoms used inside the blockade region are shaded in cyan and orange. (c) Simplified lattice for strong-coupling simulations. There is one atoms per link (encoding the spin qubit) and a double-well potential at each link (whose wells encod the position qubit); following equation (9) the relative height of the two potential wells differs by 2Δ. As spin qubits in the ground state are in, corresponding to the left (lower) well of the potential forx(y) links, the right (up) well is empty and the system is at half-filling. In order to implement equation (4), the blockade radius of the cross-controls can be limited to the first four wells around a site (shaded in cyan). Figure 3: Lattices of Rydberg atoms needed for simulating SU(2) GM. ( a ) Holographic lattice scheme for the simulation of the pure LGT at weak coupling. Blue spheres represent the control two-level atoms, whereas red spheres are the ensemble two-level atoms. The blockade radii for a plaquette-control atom and the cross-control atom are shaded in cyan and orange, respectively. ( b ) A different lattice scheme has to be used to introduce static charges. It is made from super-sites including four two-level atoms (shaded green circle). One of these is a cross-control atom (blue), whereas the other three are used to encode static charges (black). The links of the gauge magnets, which connect these effective sites, have two atoms each (red spheres on shaded green oval). Atoms used inside the blockade region are shaded in cyan and orange. ( c ) Simplified lattice for strong-coupling simulations. There is one atoms per link (encoding the spin qubit) and a double-well potential at each link (whose wells encod the position qubit); following equation (9) the relative height of the two potential wells differs by 2Δ. As spin qubits in the ground state are in , corresponding to the left (lower) well of the potential for x ( y ) links, the right (up) well is empty and the system is at half-filling. In order to implement equation (4), the blockade radius of the cross-controls can be limited to the first four wells around a site (shaded in cyan). Full size image The experiment we propose aims to detect confinement by measuring the energy of the system as a function of the distance between external charges. A linear growth of the energy is the footprint of confinement [29] . We need to prepare the ground state of the system for any g in the absence and presence of static external charges separated by different distances. We then measure the ground-state energy for each realization, obtaining its dependence on the charges separation. Before running the experiment for the full 2D GM, we propose to validate the simulator by comparing its outcomes with the known ones for the exactly solvable scenario described in the previous section, where the Hamiltonian contains only half of the plaquettes. The ground states are prepared using the adiabatic evolution implemented with the Rydberg gates (see eqaution 4). In order to apply this procedure, we need to start with a simple state with non-zero overlap with the final ground state. We also need to modify the Hamiltonian by adding that separates of more than gauge-invariant states from the non-invariant ones. At low energies, for ≫ Δ/ g , where Δ/ g is the energy scale of equation (9), the spectrum is restricted to the physical states. For example, in the validation step, the product state is a good initial state as it has non-zero overlap with of (10). Here, l h and l v are the horizontal and the vertical links of the lattice, respectively, and . Note that for the full model (9), we can use as the initial state for the adiabatic evolution, which is now performed by slowly switching on the remaining half-plaquettes [29] . The evolution is performed for a time T using the Hamiltonian H ( t )=(1− λ ( t )) H a + λ ( t )( H + H G ), with the smooth function λ ( t ) that fulfills λ (0)=0, λ ( T )=1, and H a is a gapped Hamiltonian having as a unique ground state the starting configuration. The adiabatic approximation is justified by choosing large enough compared with the inverse of the gaps of H ( t ) which stays finite during the evolution. In practice, as described in detail in Methods, the time-evolution operator is applied as a stroboscopic sequence. We divide the evolution time in a sequence of N short enough intervals δt =/ N such that , where and H I are product of Pauli matrices. Each exp( iδtλ I ( t ) H I ) can be implemented by a sequence of SRT on eight qubits (atoms), precisely, with two Rydberg gates and several single-qubit rotations ( cf . equation (4) and ref. 29 ). Even if Rydberg gates are not perfect and have a finite fidelity, the gap of the Hamiltonian and the adiabatic theorem guarantee that for large enough simulation times the final state is in the desired phase, see equation (4). The same procedure is used to obtain the ground state with two, or more, static charges. Their presence is accounted by placing new atoms on the sites of the lattice, for instance, in the lattice scheme of Fig. 3b , and enforcing equation (6) with a modified H G . In order to measure the ground-state energy of the system, we use again Rydberg gates. As discussed in Methods, they allow to map the eigenstates of each H I to states of the control atoms, which can be then read out by selective fluorescence [44] (coupling for example with a laser the state to short-lived state). Sufficient repetitions provide a measurement of the H I contribution to H . By iterating the same procedure for all the contributions H I , we can sum them up to H and measure the total energy of the system. However, a qualitative detection of the string of singlets joining the two charges, responsible of the confinement, can be done via spin-polarization spectroscopy [45] . What we have described so far is experimentally challenging but can be used to probe confinement in any regime, even away from g →0 where the confinement is expected from analytical predictions [35] . In the strongly coupled regime, the decomposition ⊗ of links makes manifest that the energy depends only on the position qubit with the state favoured (penalized) by Δ. We exploit this to design a simplified experiment based on a partial analogue encoding of links. Each spin qubit is still represented by one atom loaded in a super-lattice producing a double-well potential on each link, see Fig. 3c ). is now encoded by its position in the two wells, split by an energy 2Δ. When two static charges are added to the system, we need to introduce two extra atoms above the half-filled ground state. The creation of the strings described in the previous section can be mimicked by driving the system with , >2Δ, while simultaneously inducing in-well atom oscillations via AC-shaking [46] of the lattice at 45°. Adjusting the intensity of the shaking, we allow for the adiabatic adjustment of the atoms, which then freeze in minimal energy configurations compatible with gauge invariance. The strings can be observed by direct imaging of the atoms’ positions, for example, by joining those atoms found at the right (up) end of the x ( y ) links. This also provide the quantitative measurement of the energy needed to assess confinement. The hybrid encoding of gauge bosons allows to reduce the complexity of the simulation at the level of the digital proposal for simulating Abelian theories [29] , [37] . Contrary to the generic regime, the simplified set-up implies the existence of an upper bound on the acceptable atomic temperatures T , K B T<< Δ< . However, this condition can be satisfied in current state-of-art experiments (see equation (4)). The simulation proposed here (for similar proposals see [47] , [48] ) is only the first step towards the full quantum simulation of full-fledged QCD. Note that a slight modification of the model considered here allows for a relativistic dispersion relation as required by QCD [35] . This is only the first proposal for a generic experimental implementation of non-Abelian LGT, and as such its realization is, in its present form, very challenging. Nevertheless we do believe that this work will set the basis and serve as an inspiration for further researches that will certainly lead to simplifications and improvements. The physics we described here is dominated by the presence of singlets that have a fundamental role in high-temperature superconductivity. We foresee that the experiments we propose provide also new insights in this area (see also refs 49 , 50 ). An interesting development would be to apply the ideas of Abanin and Demler [51] and Cardy [52] to measure in the experiments the intrinsic LRE carried by a single chromo-electric string and to perform a careful analysis of other possible error sources such as atom losses. Using Rydberg gates Mesoscopic Rydberg gates are used both for the ground-state preparation and its energy measurement. The ground state for different charge backgrounds , is obtained as the ground state of a generalized Hamiltonian that include a term forcing gauge invariance, = H + H G (see main text). We start the adiabatic preparation from an easy-to-prepare unique ground state of an Hamiltonian H a , such that ≠0, for example, . During the evolution, H a is slowly substituted by , during total time T ≫ 1/Δ. In order to implement the time evolution under ( t ), we decompose it in tensor products of Pauli operators. For simplicity, let us focus just on a single plaquette. It acts on eight atoms encoding eight qubits I =( i 1 ⋯ i 8 ), and i =0, 1, 2, 3, with σ 0 =. For each H I , the plaquette state decomposes as with and . The evolution is approximated by a sequence of short steps, of a duration δt =/ N each where and ε ( I , t )= λ I ( t ) δt . The energy is measured by determining each of the as with the λ ’s from equation (11). Experimentally, we determine a single by acting with on the state ⊗ . This gives , with defined in equation (12). Up to single-qubit rotations of the ensemble qubits, is the Mesoscopic Rydberg gate responsible of the SRT on all the eight qubits conditioned on the state of the control [33] . Thus, at the price of iterating the process enough times, we can couple 0 c to a short-lived metastable state and measure by fluorescence. A single W I ( δt ) of equation (13), acting on ψ( t ) produces Experimentally, we realize it by applying the gate to ⊗ [37] . The complete experimental sequence is the following: (a) obtaining the ground state by iterative applications of the W I ( δt ) and (b) measuring each one of the H I contributions to the energy. The latter inevitably disrupts the ground state, thus, the sequence (a) and (b) needs to be repeated several times. Temperature of the atomic sample Here we discuss the effects of the environment on the temperature of the atomic sample. In full digital simulation (for mixed-analogue see Methods), thermal excitations of the atomic sample can be decoupled from GM. Indeed, the logical (hyperfine) states can be Zeeman split by an energy δE ≫ K B T . Note that by taking δE ≫ , the phase difference due to δE is quickly oscillating and cancels from the time-evolution of logic states. Furthermore, by working with a sufficiently deep optical lattice potential V 0 , we can suppress any excitation due to laser pulses, that is, the gap to the first lattice mode w can be much larger than E R , the recoil associated to Rydberg excitation, as , with , the recoil energy of lattice lasers. Note that in typical two-photon excited Rydberg nS states in Rb with n ~50 (typical pulses, 480–780 ν m ), by taking counterpropagating pulses, E R ~ E r , and ordinary values of V 0 ≳ 25 E r for Mott regime are sufficient. Thus, the real temperature of the sample is not increased by laser pulses, whose recoil energies are dispersed by the lattice itself. Thus, the digital temperature of GM is zero. Spontaneous decay of Rydberg and logical states of atoms Here we discuss how the environment affects the spontaneous decay of the Rydberg atoms. The atoms are in the Rydberg states only when the gates are working. As the typical time scale τ G needed to perform the gate is of μ s a life time τ D of tens of μs is sufficient. For the typical Rydberg states mentioned above, which can be excited relatively fast and with high fidelity (Rabi frequencies of 500 kH z with line widths of 3 kHz are realized), τ D ≳ 50 μ s , thus ≲ 10 −5 and the spontaneous decay is quite rare during the whole experiment. To conclude, we note that the coherence time, that is, the time for which the simulator can work is only limited by the life time of the metastable logical states. Such time is of order 0.1–1 s, thus in principle 10 5 –10 6 Rydberg gates can be safely applied. Fidelity of realistic Rydberg gate Here we discuss how the environment affect the fidelity of the Rydberg gate. In the main text, we have assumed that Rydberg gate to be ideal. The functioning of a realistic Rydberg gate and its fidelity were first discussed in the original paper [33] , where the major source of infidelity was re-conducted to the imperfect blockade due to the mutual interaction of two or more ensemble atoms simultaneously excited to Rydberg states. As argued in [37] , such imperfection together with possible others can be modelled as follows: where and G I was given above. We may fix the norm of operator Q I to 1 such as the parameter ϕ measures the infidelity of the gate. Some consideration on the form of Q I . We may expect that the operator decomposes in a systematic error part (which still depends on H I ), and a fluctuating random part, which is different each time the gate acts (and which we may suppose independent of H I ). Hence, we distinguish the Q I at different time with a prime (for simplicity below we omit the suffix I ). It follows that for a realistic unitary evolution, there is non-zero probability, once initialized the control in the state , of ending in . Thus, to avoid error propagation, we have to force radiative decay of the control from to , at the price that the process becomes dissipative. The evolution is where Note that the evolution is dissipative already at first order in ϕ. Indeed, and, by neglecting λ 2 terms, we have on average where represents the systematic error, which depends on the H I . Note that at first order the evolution of the system under the total Hamiltonian is simple obtained by summing over I . Thus, the infidelity of the gate has two consequences. First, we are not preparing the ground state of but of a perturbed one. However, as we are interested in a gapped phase, the adiabatic theorem ensures that the two states are very similar, so that error is only linear in ϕ for ϕ <<1. Note that ϕ depends on the efficiency of the electromagnetic-induced transparency employed in the Rydberg gate and can be about 10 −2 (ref. 33 ). The second consequence is dissipation. After the adiabatic evolution, we have a mixed state. As H I and Q have finite norm, |{ H I , }| admits one or more states which are eigenvectors with maximum eigenvalue. Thus, each dissipative term tries to drive the system to such states. As the different { H I , } are expected to be not commuting for different I , we may conjecture that their action is to drive the system to thermal state of the deformed Hamiltonian above, with a temperature of order ϕ Δ, and, thus, negligible. Strong-coupling experiment The strong-coupling scheme that we propose involves the digital simulation of only, H s ≡cross operator at site s . Owing to the analogue encoding of the position qubits of the links, each H s acts only on four atoms: thus, we have to engineer only 18 terms with Rydberg gates. The analogue encoding of the position qubit and of its dynamics has also other two consequences. First, thermal fluctuations of the atomic sample are coupled to the GM, thus, contrary to the fully digital scheme above, the absolute value of Δ and does matter. Second, the digital time corresponds to the physical time. Thus, we may estimate the highest we can engineer by identifying δt as the time employed to perform , t step . According to Trotter, . As each SRT requires two Rydberg gates, t step =18 × 2 × t R ~10 −5 s, where we assume the delay of the Rydberg gate t R ~1 μs. It follows that we can neglect the temperature T of the sample for K B T <<Δ<< ~10 −7 °K. We conclude with few comments on AC-shaking procedure. The adiabatic modulation of AC-periodic forcing of the lattice provides the hopping the atoms need to adjust to the ground state. Such hopping is controllable and selective, as it appears only if the frequency of the forcing ω is commensurable with 2Δ [53] . This avoids unwanted tunnelings as, for instance, of the control atom to the link wells and vice-versa. Next-to-nearest neighbour hoppings between different links are strongly suppressed by the exponential decay of Wannier functions. In order to induce the same rate of in-well oscillations for horizontal and vertical links, the periodic forcing F is chosen to be parallel to the plane at a 45° angle, F ||(1,1,0). How to cite this article: Tagliacozzo, L. et al . Simulation of non-Abelian gauge theories with optical lattices. Nat. Commun. 4:2615 doi: 10.1038/ncomms3615 (2013).